Hypoxia-inducible hydrogels Oxygen is vital for the existence of all multicellular organisms, acting as a signalling molecule regulating cellular activities. Specifically, hypoxia, which occurs when the partial pressure of oxygen falls below 5%, plays a pivotal role during development, regeneration and cancer. Here we report a novel hypoxia-inducible (HI) hydrogel composed of gelatin and ferulic acid that can form hydrogel networks via oxygen consumption in a laccase-mediated reaction. Oxygen levels and gradients within the hydrogels can be accurately controlled and precisely predicted. We demonstrate that HI hydrogels guide vascular morphogenesis in vitro via hypoxia-inducible factors activation of matrix metalloproteinases and promote rapid neovascularization from the host tissue during subcutaneous wound healing. The HI hydrogel is a new class of biomaterials that may prove useful in many applications, ranging from fundamental studies of developmental, regenerative and disease processes through the engineering of healthy and diseased tissue models towards the treatment of hypoxia-regulated disorders. An emerging paradigm in the mimicry of three-dimensional (3D) microenvironments involves using a variety of bioinspired materials to reconstruct critical aspects of the native extracellular niche [1] , [2] . Synthetic hydrogels have attracted substantial attention as 3D microenvironments owing to their structural similarity to the natural extracellular matrix (ECM) and their tunable properties [3] , [4] . Researchers have endeavoured to develop synthetic hydrogels to recapitulate temporal and spatial complexity in the native ECM, which varies not only in composition but also in physico-chemical parameters, including cell adhesion ligands [5] , growth factors/cytokines [6] , mechanical properties [7] , proteolytic degradability [8] and topography [9] . Thus, these studies have established how such parameters individually or synergistically regulate cell behaviour. Oxygen (dioxygen, O 2 ) is vital for the existence of all multicellular organisms, acting as a signalling molecule for cells and regulating their metabolism, survival, cell-to-cell interactions, migration and differentiation [10] , [11] . Cellular responses to O 2 deprivation (hypoxia) are primarily regulated by hypoxia-inducible factors (HIFs) that accumulate under hypoxic conditions and activate the expression of numerous genes that regulate myriad cellular activities [12] . HIFs act as key regulators, promoting angiogenesis during embryonic development, tumour progression and tissue regeneration [13] , [14] , [15] . HIFs regulate the expression of many angiogenic genes that promote vascular differentiation and morphogenesis, such as vascular endothelial growth factor (VEGF), VEGF receptor 2 (VEGFR2) [16] , [17] , [18] , angiopoietin 1 (ANG1) [19] and matrix metalloproteinases (MMPs) [20] , [21] , [22] , [23] , [24] . Although hypoxia plays a pivotal role in vascular development, nobody has simulated controlled hypoxia in a 3D microenvironment. This study reports a new class of O 2 -controlling biomaterials, hypoxia-inducible (HI) hydrogels, that can serve as 3D hypoxic microenvironments. We demonstrate control over and precise prediction of dissolved O 2 (DO) levels and gradients in the HI hydrogel. The HI hydrogel matrix stimulates tubulogenesis of endothelial-colony-forming cells (ECFCs) by activating HIFs and promotes rapid neovascularization from the host during subcutaneous wound healing. To our knowledge, this is the first hydrogel material with precisely controlled intramural DO levels, a new class of biomaterials for a wide range of possible applications. Design of HI hydrogels We began by hypothesizing that conjugating ferulic acid (FA) to a polymer backbone would let us fabricate a HI hydrogel by consuming O 2 in laccase-mediated reactions. Though many fields (for example, food chemistry and biosensors [25] ) have explored such reactions, derived from phytochemistry, they have not yet been used to fabricate O 2 controllable biomaterials. We selected gelatin (Gtn) as the polymer backbone for its cell-response properties, including cell adhesion sites and proteolytic degradability, which are critical in vascular morphogenesis [26] , [27] . Gtn would enable a relatively simple functionalization with FA for the formation of intramural hypoxia for both in vitro and in vivo vascular inductions. This approach could also generate HI hydrogels using other natural/synthetic polymers, like polyethylene glycol, hyaluronic acid and dextran. These might require incorporation of adhesion sites, such as Arg-Gly-Asp, and additional degradability features, such as MMP-sensitive peptides, depending on the application. [28] , [29] , [30] We synthesized HI hydrogels by coupling carboxyl groups of FA to amine groups of Gtn (GtnFA) via a carbodiimide-mediated reaction ( Supplementary Fig. 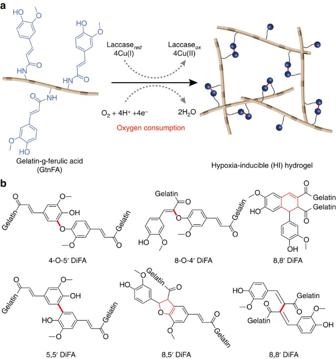Figure 1: Hypoxia-inducible hydrogel synthesis and crosslinking chemistry (a) Schematic representation of HI hydrogel formation. HI hydrogels are formed via laccase-mediated dimerization of FA molecules with O2consumption. Laccase catalyses the four-electron reduction of O2to water molecules, resulting in oxidation of FA molecules to form diferulic acid (DiFA), crosslinking the polymer networks. (b) Different chemical structures of DiFA could crosslink GtnFA polymer chains. Newly formed chemical structures are indicated in red. 1 ; Supplementary Table 1 ) and characterized the chemical structure of the functionalized polymer using 1 H NMR, indicating the specific peaks of anomeric carbon and alkyl protons of Gtn, as well as the aromatic protons of FA ( Supplementary Fig. 2a ). UV/VIS spectroscopy determined the degree of substitution (DS) of the FA molecule ( Supplementary Fig. 2b ). We fabricated the HI hydrogel by crosslinking FA molecules via a laccase-mediated chemical reaction ( Fig. 1a ) to form diferulic acid (DiFA) [31] , which yields polymer networks ( Fig. 1b ) [32] . Figure 1: Hypoxia-inducible hydrogel synthesis and crosslinking chemistry ( a ) Schematic representation of HI hydrogel formation. HI hydrogels are formed via laccase-mediated dimerization of FA molecules with O 2 consumption. Laccase catalyses the four-electron reduction of O 2 to water molecules, resulting in oxidation of FA molecules to form diferulic acid (DiFA), crosslinking the polymer networks. ( b ) Different chemical structures of DiFA could crosslink GtnFA polymer chains. Newly formed chemical structures are indicated in red. Full size image To test hydrogel formation and viscoelastic modulus, we performed rheological analysis, including dynamic time sweep of hydrogels with varying laccase concentration ( Fig. 2a–c ). The crosslink point of elastic ( G ′) and viscous ( G ″) modulus, which provides an estimate of the gelation time, occurs within 2–30 min, suggesting that laccase concentration affects the network formation kinetics. These data agree with the gelation kinetics observed by phase transition ( Fig. 2d,e ), suggesting that higher concentrations of laccase or polymer induce faster hydrogel formation. These results could have occurred because the rate of radical generation, which can induce DiFA formation, increased with higher laccase and polymer concentrations. Moreover, viscoelastic measurements showed tunable mechanical properties of the HI hydrogels (35–370 Pa), suggesting that they could maintain their 3D shapes, providing structural frameworks as extracellular microenvironments to support cell function. Another parameter to consider in designing cellular microenvironments, proteolytic degradability allows cell migration and niche remodelling [4] , [8] . Thus, we examined protease-sensitive degradation of HI hydrogels. We observed that hydrogels incubated with collagenase degraded completely within 3 h, the rate varying with the concentrations of collagenase (0.001–0.05%) and polymer (3–5%) solutions ( Fig. 2f,g ). These data demonstrate that the proteolytic degradability of the Gtn-based HI hydrogel is retained following functionalization with FA molecules. 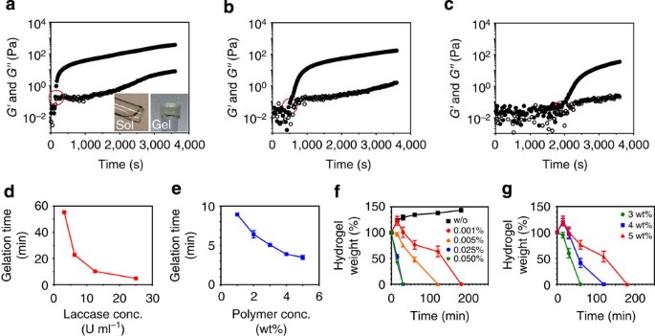Figure 2: Network formation kinetics and proteolytic degradation of HI hydrogels. Elastic modulus (G′, filled symbols) and viscous modulus (G′′, open symbols) of HI hydrogels as a function of time. Rheological analysis shows dynamic network formation and gelation kinetics for 3 wt% of HI hydrogel with laccase concentration of: (a) 25 U ml−1(inset micrographs show sol-gel transition of the hydrogels); (b) 12.5 U ml−1; and (c) 6.3 U ml−1. Measurements were performed with constant strain of 10% and frequency of 0.1 Hz using 25 mm plate. Red circles represent the cross point ofG′andG′′indicating the gelation time. Effect of (d) laccase concentration and (e) polymer concentration on gelation time. Effect of (f) collagenase concentration and (g) polymer concentration on degradability. Results ind–gare shown as the average values±s.d. (n=3). Figure 2: Network formation kinetics and proteolytic degradation of HI hydrogels. Elastic modulus ( G′ , filled symbols) and viscous modulus ( G′′ , open symbols) of HI hydrogels as a function of time. Rheological analysis shows dynamic network formation and gelation kinetics for 3 wt% of HI hydrogel with laccase concentration of: ( a ) 25 U ml −1 (inset micrographs show sol-gel transition of the hydrogels); ( b ) 12.5 U ml −1 ; and ( c ) 6.3 U ml −1 . Measurements were performed with constant strain of 10% and frequency of 0.1 Hz using 25 mm plate. Red circles represent the cross point of G′ and G′′ indicating the gelation time. Effect of ( d ) laccase concentration and ( e ) polymer concentration on gelation time. Effect of ( f ) collagenase concentration and ( g ) polymer concentration on degradability. Results in d – g are shown as the average values±s.d. ( n =3). Full size image We evaluated the cytocompatibility of hydrogels using human fibroblasts. We first examined the toxicity of the GtnFA conjugate and laccase because precursor and free enzyme molecules have the potential to induce toxicity in a hydrogel matrix. We observed no significant cytotoxicity in the GtnFA polymer and laccase (80–98% of control) ( Supplementary Fig. 3a,b ). We also encapsulated fibroblasts within the HI hydrogels to determine cell viability and morphological changes within the matrix. The results show a predominantly viable fibroblast population, as well as cell spreading and elongation within HI hydrogel matrices ( Supplementary Fig. 3c,d ). Similar viability was observed when encapsulating ECFCs ( Supplementary Fig. 3e ). We demonstrate the successful preparation of cytocompatible HI hydrogels with tunable parameters essential for their use as a 3D cellular microenvironment [2] , [4] , [33] . Controllable O 2 levels and model predictions We next hypothesized that GtnFA induces polymer network formation by O 2 consumption during hydrogel formation. To determine O 2 levels within the matrix, we monitored DO levels at the bottom of hydrogels using a noninvasive sensor patch [34] . We found that several factors—including hydrogel thickness, laccase concentrations, and DS values of polymer—affected DO levels and O 2 consumption rates. It should be noted that we used the same concentration of FA molecule, maintaining the same crosslinking density and thus diffusivity in all samples examined. Increasing laccase concentrations decreased both the DO levels and the time to reach the minimum DO level (DO min ), demonstrating that high laccase concentrations induce rapid O 2 consumption reactions and low O 2 levels ( Fig. 3a ). These data agree with the results of hydrogel formation studies, indicating that laccase concentrations significantly affect both hydrogel network formation kinetics and O 2 consumption rates. Similarly, the higher DS value of FA molecules resulted in the lowest DO levels ( Fig. 3b ). Decreasing the FA content increased the DO min . This is expected, since the FA molecule acts as a crosslinker, consuming O 2 molecules during hydrogel network formation. 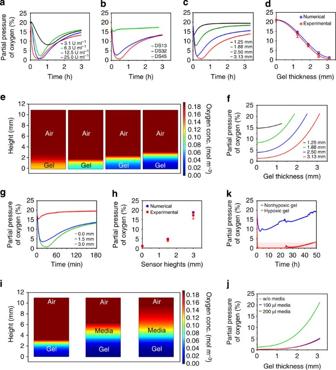Figure 3: Controlling and predicting DO levels in HI hydrogel matrix. Measured DO levels in HI hydrogels as a function of time: (a) effect of laccase concentration (3 wt%, DS 45, and 6.3−25.0 U ml−1laccase). (b) Effect of degree of substitution (DS) of FA (3 wt%, 25 U ml−1laccase and 13−45 μmol g−1of polymer). (c) Effect of hydrogel thickness (3 wt%, DS 45, and 25 U ml−1laccase) (d) Model prediction of DOminat the bottom of the HI hydrogels. We compared model numerical prediction (blue symbols) to the measured values (red symbols) to confirm the reliability of the given parameters; model predictions of DO levels and gradients after 30 min of hydrogel formation (e) in the two-layer model (air-hydrogel) and (f) across HI hydrogels, depending on different thicknesses. Formation of DO gradients within HI hydrogels (3 wt%, DS 45, and 25 U ml−1laccase) as indicated by (g) measured DO levels at different hydrogel depths as a function of time and (h) model prediction of DOminat different hydrogel depths. We compared model numerical prediction (blue symbols) to the measured values (red symbols) to confirm the reliability of the given parameters. Model predictions of DO levels and gradients after 30 min of hydrogel formation (i) in the three-layer model (air-media-hydrogel) and (j) across the HI hydrogels with the culture media. (k) DO levels of HI hydrogels encapsulated with 2 × 106cell ml−1of ECFCs as a function of hydrogel thickness (hypoxic hydrogel thickness, 2.5 mm; nonhypoxic hydrogel thickness, 1.25 mm). Results ind,hare shown as the average values±s.d. (n=3). Figure 3: Controlling and predicting DO levels in HI hydrogel matrix. Measured DO levels in HI hydrogels as a function of time: ( a ) effect of laccase concentration (3 wt%, DS 45, and 6.3−25.0 U ml −1 laccase). ( b ) Effect of degree of substitution (DS) of FA (3 wt%, 25 U ml −1 laccase and 13−45 μmol g −1 of polymer). ( c ) Effect of hydrogel thickness (3 wt%, DS 45, and 25 U ml −1 laccase) ( d ) Model prediction of DO min at the bottom of the HI hydrogels. We compared model numerical prediction (blue symbols) to the measured values (red symbols) to confirm the reliability of the given parameters; model predictions of DO levels and gradients after 30 min of hydrogel formation ( e ) in the two-layer model (air-hydrogel) and ( f ) across HI hydrogels, depending on different thicknesses. Formation of DO gradients within HI hydrogels (3 wt%, DS 45, and 25 U ml −1 laccase) as indicated by ( g ) measured DO levels at different hydrogel depths as a function of time and ( h ) model prediction of DO min at different hydrogel depths. We compared model numerical prediction (blue symbols) to the measured values (red symbols) to confirm the reliability of the given parameters. Model predictions of DO levels and gradients after 30 min of hydrogel formation ( i ) in the three-layer model (air-media-hydrogel) and ( j ) across the HI hydrogels with the culture media. ( k ) DO levels of HI hydrogels encapsulated with 2 × 10 6 cell ml −1 of ECFCs as a function of hydrogel thickness (hypoxic hydrogel thickness, 2.5 mm; nonhypoxic hydrogel thickness, 1.25 mm). Results in d , h are shown as the average values±s.d. ( n =3). Full size image Finally, we determined the influence of hydrogel thickness on DO levels. We varied gel thickness in a volume-dependent manner. Figure 3c shows that controllable DO levels depend on the HI hydrogel thickness (3 wt%, DS 45, and 25 U ml −1 laccase). The DO min decreased as thickness increased, demonstrating that intramural DO levels vary with matrix thickness. Notably, we observed DO levels within thick hydrogels (>2.5 mm) reaching hypoxic levels (<5%). To enable accurate prediction of DO levels and gradients within HI hydrogels, we employed a mathematical model developed in our previous report. [34] We assumed that O 2 consumption kinetics during hydrogel formation follows Michaelis–Menten kinetics, as shown in equation (2). To accurately estimate DO gradients in HI hydrogels, we first determined the V max and K m parameters. We measured DO levels in hydrogels (3 wt%, DS45, and 25 U ml −1 laccase) until they reached steady state. We plotted the O 2 consumption rate of the laccase-mediated reaction (experimental data) and the theoretical Michaelis–Menten equation (numerical model) using the initial V max and K m values. We then calibrated the graphs while varying the V max and K m parameters to obtain the best fit to the experimental values according to the residual sum of squares method ( Supplementary Fig. 4 ). We determined that the V max and K m values of our HI hydrogels were 0.43 μM/second and 70 μM, respectively. We then compared the experimental DO values at the different hydrogel thicknesses to numerical DO values determined by the mathematical modelling to confirm the reliability of the given parameters. As can be seen, the experimental values are similar to the numerical model simulated by using the obtained V max and K m values ( Fig. 3d ). These results showed that the O 2 consumption rate (for example, hydrogel formation kinetics) follows the theoretical Michaelis–Menten equation. Using the Michaelis–Menten parameters determined for the given conditions, we estimated the DO gradients throughout the gel depth in a two-layer (air-hydrogel) model. We found that, 30 min after hydrogel formation, the 5 DO levels at the bottom of hydrogels decreased as gel thickness increased, due to insufficient O 2 diffusion ( Fig. 3e ), and a broad range of O 2 tensions occurred within the gel matrices ( Fig. 3f ). For instance, the O 2 gradient of the thin hydrogel (1.25 mm) ranged from 15 to 17%, while a thicker one (3.13 mm) exhibited a 1.8–21% range. Measurements of DO at different hydrogel depths confirmed the accuracy of the simulation, demonstrating DO gradient throughout the hydrogel matrix ( Fig. 3g,h ) and the robust effect of hydrogel thickness on O 2 levels and gradients. Overall, O 2 measurements and computer simulations showed that our HI hydrogels consume O 2 during their formation, yielding an O 2 gradient within the matrix. Various factors could affect O 2 consumption rate and thus regulating not only the level of O 2 tensions but also the range of O 2 gradients. This is a very important advantage of the HI hydrogels as O 2 gradients are generated in many tissues during embryonic development, tissue regeneration and cancer growth [13] , [35] , [36] , [37] , [38] . Overall, the HI hydrogels may provide an innovative approach to generate hypoxic environments towards the delineation of the mechanism by which hypoxia regulates cellular responses and may facilitate the discovery of pathways involved in O 2 gradient environments. Hypoxic microenvironment for vascular tube formation We next speculated that HI hydrogel could provide controllable hypoxic environments to generate tissue models in vitro. Towards this, we selected an optimized hydrogel sample (3 wt% of polymer concentration, DS 45 of FA, and 25 U ml −1 laccase) and controlled the DO levels by altering thickness. We first performed computer simulation for media effects on O 2 gradients using a three-layer (air-media-hydrogel) model. As Fig. 3i,j shows, hydrogels placed in media for 30 min exhibited lower intramural DO levels. In fact, at thicknesses between 2.5 and 3.13 mm, DO levels were hypoxic (<5%) through the hydrogels’ depth, suggesting their potential suitability for providing artificial hypoxic microenvironments. Towards using the HI hydrogel to study vascular morphogenesis, we chose to encapsulate ECFCs, which are capable of undergoing morphogenesis in synthetic matrices [26] , [39] . We first determined how DO levels of hydrogels encapsulated with ECFCs depend on gel thickness. To test this, we encapsulated ECFCs within HI hydrogel matrices of different thickness (hypoxic gel, 2.50 mm; nonhypoxic gel (control), 1.25 mm) and cultured the constructs in ECFC media. Interestingly, the DO levels of the hypoxic gels decreased markedly for the first 30 min and retained prolonged low O 2 levels for up to 50 h ( Fig. 3k ), demonstrating that the HI hydrogel allowed the exposure of ECFCs to hypoxia and that the ECFCs also affected O 2 levels within the matrix. In fact, the DO levels of hypoxic gels without cells reached DO min within 30 min, followed by a gradual increase after the inflection point, while the DO levels within the hypoxic gels encapsulating ECFCs remained hypoxic after DO min for up to 50 h ( Fig. 3k ) due to O 2 consumption by the cells. In contrast, nonhypoxic gels exhibited higher O 2 levels (>8%) than hypoxic gels but with a similar pattern, due to the encapsulated ECFCs. We show that hypoxic environments can be generated and controlled in cultured HI hydrogels independently of cell encapsulation. Importantly, as O 2 consumption rates vary among different cell types, the HI hydrogel system provides opportunity to study hypoxia in diverse tissue models in vitro . We also show that the hypoxic environment in HI hydrogels is affected by the encapsulated ECFCs, which support continuous hypoxic environments. To study the importance of the 3D hypoxic niche in cellular response, we next hypothesized that HI hydrogels would stimulate vascular morphogenesis through HIF pathway activation. To test this, we encapsulated ECFCs within HI hydrogel matrices of different thicknesses (hypoxic gel, 2.50 mm; nonhypoxic gel (control), 1.25 mm) and cultured them for up to 3 days. We observed different cell morphologies in hypoxic versus nonhypoxic gels. Unlike the limited sprout and tube formation of ECFCs within the nonhypoxic hydrogels, ECFCs within hypoxic gels underwent tubulogenesis, forming complex network structures after 3 days in culture ( Fig. 4a ). We also found significant increases in tube coverage, length and thickness ( Fig. 4b–d ), demonstrating that our HI hydrogels stimulate vascular morphogenesis. We observed more evolved vascular structures in hypoxic gels than in nonhypoxic gels, as demonstrated by 3D z −stack confocal analysis ( Fig. 4e ). We further noticed the formation of lumens in the vascular structures formed in hypoxic hydrogels, indicating mature vascular tube formation ( Fig. 4e and Supplementary Fig. 5 ). 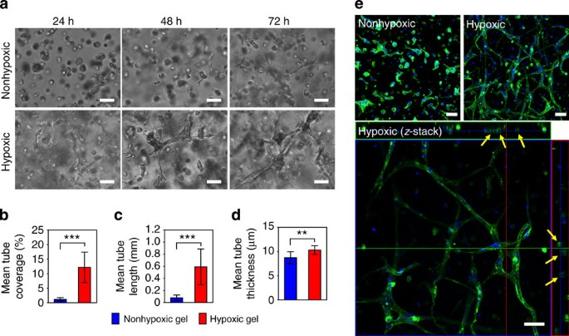Figure 4: The HI hydrogel as a dynamic microenvironment for vascular morphogenesis. Vascular tube morphogenesis by ECFCs within the HI hydrogels. (a) Light micrographic images of ECFCs encapsulated within HI hydrogels during 3 days of culture. Scale bars, 50 μm. Quantitative analysis of vascular tube formation shows (b) mean tube coverage, (c) tube length and (d) tube thickness. (e) Confocal microscopic images of ECFCs encapsulated within nonhypoxic gel and hypoxic gel; confocalz-stacks and orthogonal sections show lumen formation (indicated by arrows) within the vascular networks (phalloidin in green; nuclei in blue). Scale bars, 50 μm. Results inb–dare shown as the average values±s.d. Significance levels were set at *P<0.05, **P<0.01 and ***P<0.001. Figure 4: The HI hydrogel as a dynamic microenvironment for vascular morphogenesis. Vascular tube morphogenesis by ECFCs within the HI hydrogels. ( a ) Light micrographic images of ECFCs encapsulated within HI hydrogels during 3 days of culture. Scale bars, 50 μm. Quantitative analysis of vascular tube formation shows ( b ) mean tube coverage, ( c ) tube length and ( d ) tube thickness. ( e ) Confocal microscopic images of ECFCs encapsulated within nonhypoxic gel and hypoxic gel; confocal z -stacks and orthogonal sections show lumen formation (indicated by arrows) within the vascular networks (phalloidin in green; nuclei in blue). Scale bars, 50 μm. Results in b – d are shown as the average values±s.d. Significance levels were set at * P <0.05, ** P <0.01 and *** P <0.001. Full size image To better understand the molecular mechanisms underlying tube formation in HI hydrogels, we analysed relevant gene expression soon after ECFC encapsulation. We found that ECFCs cultured in hypoxic gels expressed significantly higher levels of two isoforms of HIFα (HIF-1α and HIF-2α) after 12 h than ECFCs within nonhypoxic hydrogels ( Fig. 5a ). Interestingly, we found that HIF-1α gene expression gradually became upregulated in ECFCs in nonhypoxic gel for up to 24 h during the culture period, probably due to the presence of FA molecules. A recent study demonstrated that free FA molecules could induce upregulation of HIF-1α expression in endothelial cells (ECs) in a concentration-dependent manner [40] . We also examined the expression of three MMP genes in ECFCs—membrane type 1 (MT1)-MMP, MMP-1 and MMP-2—as these play a critical role in vascular morphogenesis [26] , [41] , [42] . We found that all MMP gene expressions in ECFCs from the hypoxic gel were upregulated over 48 h of culture compared with ECFCs encapsulated in non-hypoxic gel ( Fig. 5b ). We also confirmed protein levels and activities, finding higher levels of MT1-MMP and activated forms of MMP-1 and MMP-2 in hypoxic hydrogels ( Supplementary Fig. 6 ). Finally, we examined the gene expression of proangiogenic factors within the hypoxic microenvironment. We noticed upregulation of VEGF and VEGFR2 in ECFCs encapsulated in hypoxic gels compared with nonhypoxic gels ( Fig. 5c ). ANG1 , which contributes to blood vessel maturation and stabilization, was upregulated, while ANG2 , an antagonist of ANG1 , was downregulated in hypoxic hydrogels compared with nonhypoxic hydrogels. ( Fig. 5c ). Collectively, these results demonstrate that hypoxic hydrogels stimulate upregulation of proangiogenic and MMP genes affecting vascular morphogenesis. 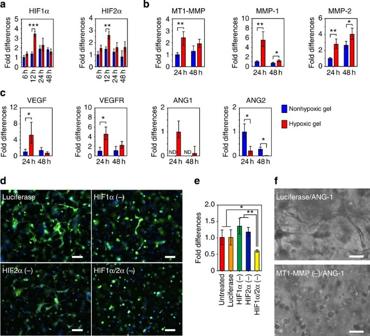Figure 5: Molecular pathway activation of vascular morphogenesis within HI hydrogels. Real-time RT-PCR analysis of gene expression of ECFCs encapsulated within the different hydrogel types: (a) HIFs, (b)MMPgenes and (c)angiogenicgenes. (d) Inhibition of vascular morphogenesis of ECFCs by siRNA HIFs suppression. Fluorescence microscopic images after 3 days in culture show that siRNA suppression of HIF-1αand/or HIF-2α affects vascular morphogenesis. Scale bars, 50 μm. (e) Real-time RT-PCR analysis ofMT1-MMPgene expression of ECFCs treated with HIF-1α and/or HIF-2α siRNA and encapsulated within the HI gel after 24 h of culture. (f) Inhibition of vascular morphogenesis of ECFCs by siRNA MT1-MMP suppression. Light microscopy images after 3 days in culture show that siRNA suppression of MT1-MMPs affect vascular morphogenesis. Scale bars, 25 μm. Results ina–c,eare shown as the average values±s.d. Significance levels were set at *P<0.05, **P<0.01 and ***P<0.001. Figure 5: Molecular pathway activation of vascular morphogenesis within HI hydrogels. Real-time RT-PCR analysis of gene expression of ECFCs encapsulated within the different hydrogel types: ( a ) HIFs, ( b ) MMP genes and ( c ) angiogenic genes. ( d ) Inhibition of vascular morphogenesis of ECFCs by siRNA HIFs suppression. Fluorescence microscopic images after 3 days in culture show that siRNA suppression of HIF-1 α and/or HIF-2α affects vascular morphogenesis. Scale bars, 50 μm. ( e ) Real-time RT-PCR analysis of MT1-MMP gene expression of ECFCs treated with HIF-1α and/or HIF-2α siRNA and encapsulated within the HI gel after 24 h of culture. ( f ) Inhibition of vascular morphogenesis of ECFCs by siRNA MT1-MMP suppression. Light microscopy images after 3 days in culture show that siRNA suppression of MT1-MMPs affect vascular morphogenesis. Scale bars, 25 μm. Results in a – c , e are shown as the average values±s.d. Significance levels were set at * P <0.05, ** P <0.01 and *** P <0.001. Full size image To further understand the pathway activation that stimulates vascular morphogenesis within the HI hydrogels, we first performed a reoxygenation study. Reoxygenation, the phenomenon in which hypoxic regions become more exposed to O 2 by changing partial pressure of O 2 , induces production of reactive O 2 specimens, which involves an angiogenic response [43] . Our previous study demonstrated that reoxygenation affected the tube formation kinetics of ECs encapsulated in collagen gels in atmospheric conditions through a HIFα-independent pathway [34] . In our HI hydrogel system, we observed slight O 2 fluctuations (from 0.1 to 1.3% O 2 ) and a gradual increase after media changes (see Fig. 3k ). Thus, we wondered whether this slight reoxygenation due to media change affects vascular morphogenesis in the HI hydrogels. We encapsulated ECFCs within HI hydrogels and cultured them for up to 3 days with or without media changes. We found that ECFCs cultured without media changes underwent vascular morphogenesis similar to those cultured with media changes ( Supplementary Fig. 7 ), demonstrating that reoxygenation does not affect the vascular morphogenesis of ECFCs in HI hydrogel systems. These results demonstrate that in contrast to existing hydrogel systems, which may provide uncontrolled and transient hypoxic environments, the HI hydrogel supports controllable and stable environments to activate hypoxia-regulated pathways. We next aimed to determine whether vascular morphogenesis within HI hydrogels occurs through the activation of HIFs. Small interfering RNA (siRNA) studies examined the involvement of HIF-1α and HIF-2α during ECFC tubulogenesis in HI hydrogels. We encapsulated ECFCs treated with either or both HIF siRNAs in HI hydrogels after confirming the suppression ( Supplementary Fig. 8 ). Knocking down each or both HIFs reduced tube formation compared with untreated and luciferase-treated ECFCs ( Fig. 5d and Supplementary Fig. 9 ). Notably, when both HIFs were knocked down, most of the encapsulated ECFCs exhibited round shapes, even after 3 days in culture ( Supplementary Fig. 9 ). To delineate whether vascular network formation in the HI hydrogel is regulated through HIF-secreted angiogenic growth factors, we examined the exogenous addition of Ang1 to the culture media (that already contains VEGF). We found that addition of Ang1 did not promote vascular network formation in the nonhypoxic hydrogels ( Supplementary Fig. 10 ). Examining MT1-MMP, we detected significant downregulation of MT1-MMP expression after 24 h of culture in the ECFCs treated with both HIFs siRNA compared with non-treated, luciferase-treated and each HIF-treated-alone groups ( Fig. 5e ). When MT1-MMP was suppressed, encapsulated ECFCs did not generate vascular networks in HI hydrogels ( Fig. 5f ; Supplementary Fig. 11 ). Collectively, these results demonstrate that accumulation of HIF-1α and HIF-2α activates MT1-MMP, which enables vascular morphogenesis of ECFCs within HI hydrogels. Indeed, MT1-MMP was previously established as a critical component for the progression of 3D tubulogenesis within hydrogel materials [26] , [41] , [42] . In sum, our HI hydrogels, which can induce hypoxic microenvironments, promote complex and mature vascular tube structures by activating HIFs through the upregulated expression of proangiogenic factors and MMPs. In vivo angiogenic effect of HI hydrogels Although numerous studies have suggested that hypoxia stimulates blood vessel formation both in vitro and in vivo [11] , [23] , [44] , nobody has yet reported inducing acute hypoxia by manipulating a material-tissue interface to affect blood vessel invasion. To investigate the potential in vivo application of HI hydrogels, we hypothesized that our hypoxic hydrogel would induce acute hypoxia in surrounding tissues through in situ gel formation with O 2 consumption, which in turn would stimulate blood vessel invasion. We first performed a simulation to estimate DO levels after in vivo injection of hypoxic hydrogels using the given parameters. For this purpose, we assumed a partial pressure of O 2 in rat subcutaneous tissue of 40 mm Hg, following previous reports [45] , [46] , although the exact pressure was not defined. We found that the DO gradient from the center of the hydrogel to the hydrogel’s edge (that is, the interface of the hydrogel and the surrounding tissue) is independent of the shape of the hydrogel ( Fig. 6a–c ). Notably, we found that DO levels at the edge of the hydrogel are lower than the physiological or pathological O 2 levels of the in vivo environments (from 10 mm Hg to 40 mm Hg; Fig. 6d–f ), suggesting that HI hydrogels can induce an acutely hypoxic environment and may stimulate the surrounding tissues. 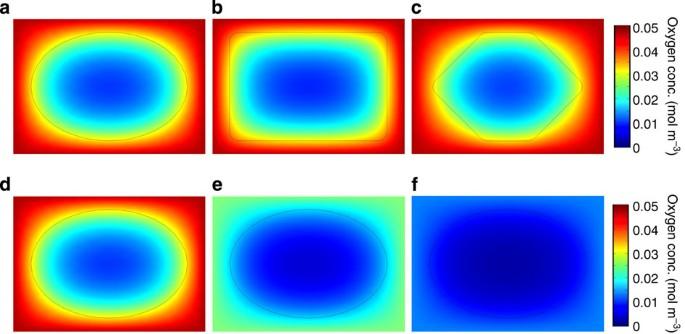Figure 6: Model prediction of DO levels in dynamicin vivoenvironments. DO gradients within the HI hydrogels after 30 min of injection depending on their shape; (a) eclipse, (b) rectangle and (c) polygonal shapes. DO gradients within the HI hydrogels after 30 min of injection depending on different surrounding O2tensions, (d) 40 mm Hg (DO levels of the hydrogel core, 8.4 × 10−3mol m−3; DO levels of the interface, 3.2 × 10−2mol m−3), (e) 20 mm Hg (DO levels of the hydrogel core, 4.2 × 10−3mol m−3; DO levels of the interface, 1.7 × 10−2mol m−3) and (f) 10 mm Hg (DO levels of the hydrogel core, 2.0 × 10−3mol m−3; DO levels of the interface, 0.8 × 10−2mol m−3). Figure 6: Model prediction of DO levels in dynamic in vivo environments. DO gradients within the HI hydrogels after 30 min of injection depending on their shape; ( a ) eclipse, ( b ) rectangle and ( c ) polygonal shapes. DO gradients within the HI hydrogels after 30 min of injection depending on different surrounding O 2 tensions, ( d ) 40 mm Hg (DO levels of the hydrogel core, 8.4 × 10 −3 mol m −3 ; DO levels of the interface, 3.2 × 10 −2 mol m −3 ), ( e ) 20 mm Hg (DO levels of the hydrogel core, 4.2 × 10 −3 mol m −3 ; DO levels of the interface, 1.7 × 10 −2 mol m −3 ) and ( f ) 10 mm Hg (DO levels of the hydrogel core, 2.0 × 10 −3 mol m −3 ; DO levels of the interface, 0.8 × 10 −2 mol m −3 ). Full size image To confirm the effect of HI hydrogels on blood vessel recruitment in vivo , we generated two types of HI hydrogels (hypoxic and nonhypoxic). To control O 2 levels in vivo , we mixed calcium peroxide (CaO 2 ) as an O 2 -releasing compound to generate nonhypoxic gels (>8% O 2 ). To generate a hypoxic gel, we encapsulated calcium hydroxide—Ca(OH) 2 —a side product of CaO 2 decomposition that does not influence the change of O 2 tension within the gel matrix ( Supplementary Fig. 12 ). We injected the hydrogels subcutaneously to mice and examined them for up to 5 days. While microvasculature was observed surrounding both hydrogels, higher density and larger size of microvasculature were observed surrounding the hypoxic hydrogel than surrounding nonhypoxic gels after 1 day. After 3 and 5 days, the density of blood vessels surrounding and penetrating the hypoxic matrices increased to a greater extent than in nonhypoxic hydrogels ( Fig. 7a–d ). Similar trends were observed in subcutaneous injections into rats ( Supplementary Fig. 13 ). Evaluating whether the recruited blood vessels are anastomosed with the host vessels and are functional, we found that within 3 days hypoxic hydrogels were invested with perfused microvasculature networks, while isolated occasions of perfused microvasculature were detected in the nonhypoxic matrices ( Fig. 8a ) These perfused networks extended throughout the entire hypoxic hydrogels after 5 days while were limited in the nonhypoxic hydrogels ( Fig. 8b ). 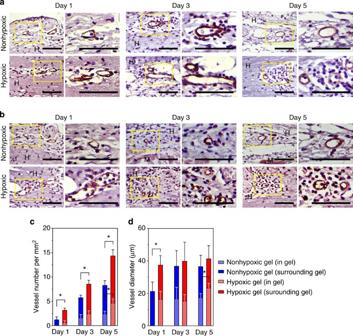Figure 7:In vivoangiogenic effect of the HI hydrogels. Histological sections of hydrogels 1, 3 and 5 days after injection stained with (a) α-SMA and (b) CD31. Right panel represents high-magnification images of the boxed regions. Quantification of blood vessels number (c) and diameter (d) surrounding and penetrating into the hydrogels. M, Muscle; H, hydrogels. Results inc,dare shown as the average values±s.d. Significance levels were set at: *P<0.05, **P<0.01 and ***P<0.001. Scale bars, 100 μm. Figure 7: In vivo angiogenic effect of the HI hydrogels. Histological sections of hydrogels 1, 3 and 5 days after injection stained with ( a ) α-SMA and ( b ) CD31. Right panel represents high-magnification images of the boxed regions. Quantification of blood vessels number ( c ) and diameter ( d ) surrounding and penetrating into the hydrogels. M, Muscle; H, hydrogels. Results in c , d are shown as the average values±s.d. Significance levels were set at: * P <0.05, ** P <0.01 and *** P <0.001. Scale bars, 100 μm. 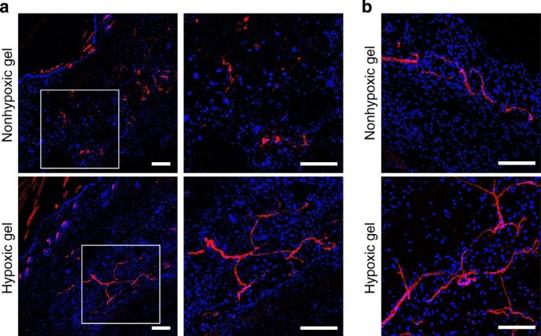Figure 8: Blood vessel perfusion within the HI hydrogels. Perfused blood vessels infiltrated into hydrogel matrix (a) 3 days and (b) 5 days after injection.GS-IB4lectin in red and nucluei in blue. Scale bars, 100 μm. Full size image Figure 8: Blood vessel perfusion within the HI hydrogels. Perfused blood vessels infiltrated into hydrogel matrix ( a ) 3 days and ( b ) 5 days after injection. GS-IB4 lectin in red and nucluei in blue. Scale bars, 100 μm. Full size image Taken together, our results demonstrate that acute hypoxic conditions induced in vivo by the HI hydrogel promote blood vessel recruitment and neovascularization from the host during the wound-healing process. Thus, HI hydrogels can be further explored as an acellular matrix for the study of hypoxia-regulated cellular processes. In addition, HI hydrogels can be delivered through injection into the site of interest, thus requiring the use of minimally invasive techniques. The current study presents a new class of synthetic biomaterials that can mimic hypoxic conditions in native niches. Our novel approach demonstrated that HI hydrogels form via an enzyme-mediated reaction with O 2 consumption. We can accurately predict and control O 2 levels and gradients within our HI hydrogels, thus offering controllable and stable hypoxic environments. ECFCs encapsulated within HI hydrogel undergo morphogenesis and generate extensive vascular network structures via HIF-mediated activation of MT1-MMP. Hypoxic hydrogels promote blood vessel recruitment and infiltration via the material-tissue interface. To our knowledge, this is the first example of HI hydrogel materials. Moreover, this approach can be adapted for many other natural/synthetic polymers and may encourage innovation in a broad range of applications, including the study and treatment of hypoxia-regulated disorders, generation of artificial tissue constructs using progenitor or stem cells in regenerative medicine and development of engineered de novo disease models such as in vitro cancer models. Materials Gelatin (Gtn, type A from porcine skin, less than 300 bloom), laccase (lyophilized powder from mushroom, ⩾ 4.0 units/mg), 3-methoxy-4-hydroxycinnamic acid (ferulic acid, FA), N -(3-dimethylaminopropyl)- N′ -ethylcarbodiimide hydrochloride (EDC), N -hydroxysuccinimide (NHS), dimethyl sulfoxide (DMSO), deuterium oxide (D 2 O) and collagenase type IV were purchased from Sigma-Aldrich (Saint Louis, MO) and used as obtained without purification. Dulbecco’s Phosphate-Buffered Saline (DPBS), Dulbecco’s Modified Eagle Medium (DMEM), and fetal bovine serum (FBS) were all purchased from Gibco, Invitrogen (Life Technologies, CA). Dialysis membrane (molecular cutoff=3,500 Da) was purchased from Spectrum Laboratories (Rancho Dominguez, CA). Synthesis of gelatin- g -ferulic acid Gelatin- g -ferulic acid (GtnFA) conjugate was synthesized using EDC and NHS as coupling reagents. For the synthesis, a mixture of DMSO and distilled water (DIW) with a 1:1 volume ratio was prepared as a solvent. Gtn (1.0 g) was dissolved in 50 ml of the solvent at 40 °C. FA (0.78 g, 4.0 mmol) was dissolved in 20 ml of the solvent and reacted with EDC (0.92 g, 4.8 mmol, 1.2 equation of carboxyl unit of FA) and NHS (0.64 g, 5.6 mmol, 1.4 equation of carboxyl unit of FA) at room temperature for 15 min to activate the terminal carboxyl groups of FA. The activated solution was then applied to the Gtn solution, and a conjugative reaction was conducted at 40 °C for 24 h. After reaction, the solution was dialysed against water for 5 days (molecular weight cutoff=3,500 Da). After dialysis, we obtained GtnFA by freeze-drying and kept the product in a refrigerator before use. The degree of substitution (DS) of FA was measured using a UV/Vis spectrometer (SpectraMax; Molecular Devices, Sunnyvale, CA). GtnFA polymer (10 mg) was dissolved in 1 ml of a mixture of DMSO and DIW with a volume ratio of 1:1, and the absorbance was measured at the 320 nm wavelength. The concentration of the conjugated FA molecules was calculated from a calibration curve given by monitoring the absorbance of a known concentration of FA; it was standardized with the baseline measured using Gtn solution (10 mg ml −1 ). The chemical structure of GtnFA was characterized using a 1 H NMR spectrometer (Bruker AMX-300 NMR spectrometer, Billerica, MA). The GtnFA polymer solution (10 mg ml −1 of D 2 O) was prepared for the measurement. Supplementary Table 1 lists the synthesized polymer series depending on the feed amount of FA molecules. Preparation of hypoxia-inducible hydrogels Hypoxia-inducible (HI) hydrogels were prepared by mixing aqueous GtnFA polymer and laccase solution. Hydrogels (100 μl) were prepared in 1 ml vials at 37 °C. Seventyfive microliters of the GtnFA polymer solution (4.0–6.7 wt%) and 25 μl of laccase solution (25–100 U ml −1 of stock solution) were simply mixed and gently shaken. To generate gel matrices of different thicknesses, we fabricated HI hydrogels in a 96-well plate (BD Bioscience or DO sensor patched plate-please see below for details) in a volume-dependent manner. For example, to generate hydrogel that was 2.5 mm thick, we pipetted 80 μl of the mixture of polymer and laccase solutions in each well and allowed them to react at 37 °C. All solutions used were dissolved in DPBS (pH 7.4), and the final concentration of the hydrogels was 3–5 wt%. Gelation time The gelation time of the HI hydrogels was determined by the vial-tilting method [47] . We prepared 100 μl of hydrogel in a 1-ml vial and mixed gently to initiate the crosslinking reaction at 37 °C. Gelation time was measured as the time point after inverting the solution when more than 3 min passed without flow. The experiments were performed with different concentrations of laccase and polymer, as detailed in the article. Measurement of viscoelastic properties We performed rheological analysis of the HI hydrogels using a rheometric fluid spectrometer (RFS3, TA Instruments, New Castle, DE) with a 25 mm plate geometry. In the rheological experiments, hydrogel samples were prepared on the plate in the instrument. We performed dynamic time sweeps on hydrogel samples in various conditions. We monitored the elastic modulus ( G′ ) and viscous modulus ( G′′ ) at 10 percent of strain and a frequency of 0.1 Hz at 37 °C. A solvent trap wetted with deionized water was used to prevent sample evaporation. In vitro proteolytic degradation study In vitro degradation of HI hydrogels was gravimetrically determined. Hydrogels (100 μl) were prepared in microtubes and subsequently incubated in 500 μl of PBS with or without collagenase at 37 °C. We removed the media from the microtubes at a pre-determined time and measured the weight of degraded hydrogels ( W d ). Fresh media were added into the tube after weighing. The weight of the remaining hydrogels was then calculated according to the following equation (1): where W d is the weight of the degraded hydrogels and W i is the weight of the initial hydrogels. Cytocompatibility of HI hydrogels All solutions for the in vitro cytotoxicity and viability studies were prepared using DPBS and filtered for sterilization using a syringe filter with a pore size of 0.2 μm. We investigated the cytotoxicity of the synthesized polymer and the enzyme using XTT (Sigma-Aldrich), according to the manufacturer’s instructions and our previous report [48] . In brief, newborn human foreskin fibroblasts (NUFF; Global Stem, Rockville, MD) were expanded. To test cytocompatability, 2.8 × 10 4 cells cm −2 were cultured in 100 μl media and in the presence of polymer solution (0.63–10.0 mg ml −1 ) or laccase solution (1.6–25 U ml −1 ) for 24 h, following by their incubation in medium containing 20 percent (v/v) XTT solution for 4 h. For the quantitative analysis, we removed 100 μl of the medium, placed it in a 96-well plate and read it in a microplate reader at the 450 nm wavelength. Cell viability was determined as a percentage of control cells (nontreated cells that were defined as 100% viable). Cell viability of HI hydrogels was evaluated using a live/dead kit (Invitrogen). In brief, 5 × 10 5 NUFF cells ml −1 were encapsulated within HI hydrogels and cultured under standard cell culture conditions (37 °C and 5% CO 2 ) in high-glucose DMEM with 10% FBS. After incubation for 2 and 24 h, we treated each well with 100 μl of 2 μM of the acetomethoxy derivate of calcein (calcein AM) and 4 μM of ethidium homodimer-1 (EthD-1) mixture and incubated at 37 °C for 30 min. The stained samples were washed three times using PBS and then counted with fluorescence microscopy (BX60, Olympus, Tokyo, Japan). DO measurement and mathematical model prediction We measured DO levels non-invasively throughout hydrogels using commercially available sensor patches (Presens, Regensburg, Germany), as previously described [34] , [49] , [50] . To measure O 2 levels at the bottom of hydrogels, the polymer solutions were added on top of the sensors, which were immobilized in each well of a 96-well plate (BD Bioscience), and then mixed with laccase solutions. To measure O 2 levels within different regions of the hydrogel (top, 3 mm; middle, 1.5 mm), we measured O 2 levels using a simple device we designed ( Supplementary Fig. 14 ). All experiments were conducted in a controlled environment at 37 °C and 5% CO 2 in incubators with and without culture media (DMEM plus 10% FBS). We controlled hydrogel thicknesses by varying the solution volume. DO gradients within the hydrogels were estimated using a mathematical model based on Michaelis–Menten kinetics, as described in our previous report [34] . In brief, we assumed that the O 2 consumption rate ( R ) of laccase-mediated crosslinking reactions follow Michaelis–Menten kinetics (equation 2) and determined the Michaelis–Menten parameters of the O 2 -consuming hydrogel formation. where V max represents the maximum O 2 consumption rate and K m is the O 2 concentration at which the reaction rate is half of V max . To determine these parameters, we measured the steady-state DO level of 3 wt% hydrogel (DS 45) formed with 25.0 U ml −1 laccase and plotted the experimental data using the Michaelis–Menten equation. We also calibrated the plots according to the residual sum of squares method to give the best-fit graphs between the theoretical equation and experimental values. We simulated the two-layer (air-hydrogel) and three-layer (air-media-hydrogel) models of the DO gradients with commercial software, Comsol Multiphysics (Comsol, LA, CA), as previously described [51] . ECFC encapsulation and viability All solutions for the in vitro viability were prepared using DPBS and filtered for sterilization using a syringe filter with a pore size of 0.2 μm. ECFCs (Lonza, Walkersville, MD) were cultured, as previously described [52] , in endothelial growth media-2 (EGM2; Lonza) containing VEGF and 10% FBS on the plate coated with type I collagen (BD Biosciences, Franklin Lakes, NJ). GtnFA polymer solution (4 wt%) was dissolved in PBS (pH 7.4) and mixed with ECFC pellets to provide cell suspension, and then laccase solution (100 U ml −1 ) was added at a volume ratio of 3:1 (polymer solution:laccase solution) and gently mixed for 2 min at 37 °C. The final concentration of the polymer, laccase and cells were 3 wt%, 25 U ml −1 and 2 × 10 6 cells ml −1 , respectively. The mixture was placed in the 96-well plate and allowed to react at 37 °C for 15 min. The ECFCs encapsulated within the hydrogels were cultured with 200 μl in growth media (Lonza) under standard cell culture conditions (37 °C and 5% CO 2 ) for up to 72 h. The culture medium was replaced every 24 h. For viability, after incubation for 24 and 72 h, we treated each well with 100 μl of 2 μM of calcein AM and 1 μM of EthD-1 mixture, incubate and analysed as detailed above for NUFF cells. We observed the ECFCs at different region of hydrogels by controlling the coaxial coarse/fine-focusing knob of microscope. ECFC morphologies were observed using optical microscopy (in phase-contrast mode) and confocal microscopy (LSM 510 Meta, Carl Zeiss). For confocal observations, ECFCs within hydrogels were fixed using 3.7% paraformaldehyde for 40 min at room temperature and washed three times using PBS. The fixed cells were permeabilized with 0.1% Triton X-100 for 20 min and incubated with 1% BSA blocking solution at room temperature for 1 h. The hydrogel samples were incubated with phalloidin (1:40; Molecular Probes, Eugene, OR) and Hoechst 33258 (1:10,000; Molecular Probes) to visualize the cytoplasm and nuclei, respectively. Real-time RT-PCR Quantitative real time RT-PCR was performed as described previously [26] , [52] . In brief, total RNA was isolated from ECFCs encapsulated in hydrogels using TRIzol (Invitrogen) according to the manufacturer’s instructions. Total RNA was quantified using an ultraviolet spectrophotometer and validated for having no DNA contamination. RNA (1 μg per sample) was transcribed using reverse transcriptase M-MLV and oligo(dT) primers (both from Promega, Madison, WI) according to the manufacturer’s instructions. We used TaqMan Universal PCR MasterMix and Gene Expression Assay (Applied Biosystems, Foster City, CA) according to the manufacturer’s instructions for HIF-1α, HIF-2α, VEGF, VEGFR, ANG1, ANG2, MT1-MMP, MMP-1, MMP-2 - and β-actin , as described previously. Live staining and angiogenesis assay We performed live staining using Calcein-AM (Invitrogen) to quantify the mean tube coverage, length and thickness, as described previously [34] . In brief, ECFCs were encapsulated and cultured for 3 days using the above-described method. One hundred microlitres of 2 μM calcein solution was added to each well, and the ECFCs embedded in the hydrogel were incubated at room temperature for 60 min. The stained cells were washed three times using PBS and then observed with fluorescence microscopy (BX60, Olympus, Tokyo, Japan). For the angiogenesis analysis, we use 5–20 images at × 20 magnifications of different fields within the hydrogels, and the vascular tube structure was analysed using MetaMorph software (Universal Imaging, Downingtown, PA) with the angiogenesis tools. Effect of ANG-1 on ECFC vascular morphogenesis in HI hydrogels We encapsulated ECFCs within HI hydrogels (hypoxic versus nonhypoxic gel) as described above and cultured them in EGM2 (Lonza) containing 10% FBS with additional 50 ng ml −1 of ANG-1. ECFC morphologies were observed using optical microscopy (in phase-contrast mode) along the 3-day culture period. Zymography We collected the conditioned media from each condition at pre-determined time points and analszed for MMP-1 and MMP-2 as previously described [39] . In brief, collected media were loaded on 10% gelatin (for MMP-2) and 12% casein (for MMP-1) zymography gels (Bio-Rad, Hercules, CA). We performed electrophoresis for 90 min at room temperature. After washing the gels in water, SDS was extracted from the gels with renaturation buffer (Invitrogen). MMP activities were developed in a developing buffer (Invitrogen) at 37 °C for 24 h and visualized by staining with Coomassie Blue R-250. Western blot We performed western blot analysis as described previously [52] . Cell lysates were prepared in a Tris-Triton-X buffer (1% Trion-X, 150 mM NaCl, and 50 mM Tris, pH 7.5) with 1 × protease inhibitor cocktail (Thermo Scientific, Waltham, MA). Protein isolated from cell lysates was quantified with the DC assay (Bio-Rad) and boiled at 95 °C for 5 min in Laemmli buffer (Bio-Rad) with β-mercaptoethanol. Protein (25 μg per well) was loaded into a 4–20 percent SDS-PAGE gel (Bio-Rad). Proteins were transferred to nitrocellulose membranes, blocked in three percent nonfat milk for 1 h, and incubated overnight at 4 °C (under constant shaking) with primary antibody: rabbit anti-MMP14 (MT1-MMP, 1:1,000) and GAPDH (1:3,000; both from Abcam, Cambridge, MA). We washed the membranes three times in Tris-buffered saline containing 0.1% Tween 20 (TBST) for 15 min each and incubated with anti-rabbit horseradish peroxidase (HRP) (1:1,000; Cell Signaling Technology, Danvers, MA). Membranes were washed three times in TBST, developed with enhanced chemiluminescence (Pierce) and visualized using the ChemiDoc XRS+ System (Bio-Rad). Small interfering RNA transfection ECFCs were transfected with siGENOME SMARTpool human HIF-1α, HIF-2 α and MT1-MMP (Dharmacon, Lafayette, CO) following the manufacturer’s protocol, as previously described [26] , [51] , [52] . Cells were seeded on a six-well plate and treated with 100 nM siRNA. We performed mRNA analysis after 24 h and used confirmed transfected cells for experiments after 48 h. In vivo subcutaneous injection We performed subcutaneous injection in rats ( n =6, 6–10 week-old Sprague–dawley female) or mice ( n =4, 6–10 week-old C57/6 female) to investigate the in vivo angiogenic effects of HI hydrogels. To control O 2 levels in vivo , we mixed a small amount of calcium peroxide (CaO 2 ; Sigma-Aldrich) and calcium hydroxide—Ca(OH) 2 (Sigma-Aldrich)—with the polymer solution. The solid calcium peroxide begins to decompose and release O 2 molecules when in contact with water [53] . Thus, we encapsulated CaO 2 as an O 2 -releasing compound to generate nonhypoxic hydrogel as a control group. To minimize the difference between the sample groups, we also encapsulated Ca(OH) 2, a by-product of CaO 2 decomposition, within hypoxic hydrogels. Ca(OH) 2 does not influence the change of O 2 tension within the gel matrix. In our initial study, we optimized concentrations of calcium derivatives to control O 2 levels for in vivo studies. We injected 200 μl of hydrogels formed with 0.02% Ca(OH) 2 (hypoxic hydrogel), and the same volume of hydrogels formed with 0.02% CaO 2 (nonhypoxic hydrogel) into the backs of animals. For this study, polymer solutions were sterilized by filtering using syringe filter (pore size, 0.2 μm) and injected using 26-gauge needles. At each pre-determined time point (1, 3 and 5 days), we killed the animals, removed the hydrogels with the surrounding tissue, fixed the explants in formalin-free Accustain fixative and proceeded to histological analysis. To confirm the vascular functionality of blood vessels infiltrated into hydrogel matrix, we injected Alexa Fluor 568-conjugated isolectin GS-IB4 from Griffonia simplicifolia (Invitrogen) through the tail veins of the mice, as we previously described [54] . After 30 min, we killed the mice, removed the hydrogels, stained with Hoechst and then proceeded for visualization using confocal microscopy (LSM 510 Meta, Carl Zeiss). The animal study was performed using a protocol (RA11A196 and MO12A210) approved by The Johns Hopkins University Institutional Animal Care and Use Committee. Histological analysis After we fixed the explants as described above, the samples were then dehydrated in graded ethanol (80–100%), embedded in paraffin, serially sectioned using a microtome (5 μm) and stained with either haematoxylin and eosin (H&E) or underwent immunohistochemistry for α-SMA and CD31. Statistical analysis We performed all measurements of hydrogel characterizations, including gelation time, proteolytic degradation and mechanical strength, using triplicate samples for each data point. We performed RT-PCR analysis for HIFs, MMPs and proangiogenic factors in triplicate with duplicate readings. We performed statistical analysis using GraphPad Prism 4.02 (GraphPad Software Inc., La Jolla, CA). We also used this software to perform t -tests to determine significance. Significant levels, determined using post-tests, were set at: * P <0.05, ** P <0.01 and *** P <0.001. All graphical data were reported. How to cite this article: Park, K. M. and Gerecht, S. Hypoxia-inducible hydrogels. Nat. Commun. 5:4075 doi: 10.1038/ncomms5075 (2014).